Epigenetic silencing ofmiR-210increases the proliferation of gastric epithelium during chronicHelicobacter pyloriinfection Persistent colonization of the gastric mucosa by Helicobacter pylori (Hp) elicits chronic inflammation and aberrant epithelial cell proliferation, which increases the risk of gastric cancer. Here we examine the ability of microRNAs to modulate gastric cell proliferation in response to persistent Hp infection and find that epigenetic silencing of miR-210 plays a key role in gastric disease progression. Importantly, DNA methylation of the miR-210 gene is increased in Hp-positive human gastric biopsies as compared with Hp-negative controls. Moreover, silencing of miR-210 in gastric epithelial cells promotes proliferation. We identify STMN1 and DIMT1 as miR-210 target genes and demonstrate that inhibition of miR-210 expression augments cell proliferation by activating STMN1 and DIMT1 . Together, our results highlight inflammation-induced epigenetic silencing of miR-210 as a mechanism of induction of chronic gastric diseases, including cancer, during Hp infection. Chronic inflammation is a critical risk factor for various types of cancer and has been estimated to cause 20% of all human cancers [1] . Specific pathogens have been identified as causal risks for particular types of cancer; Helicobacter pylori (Hp) in gastric cancer, hepatitis B and C viruses in liver cancer, papilloma virus for ovarian cancer, Eptein–Barr virus for malignant lymphoma, adult T-cell leukaemia virus for adult T-cell leukaemia and human herpes virus 8 for Kaposi’s sarcoma [2] . However, the molecular mechanisms by which these microbial infections trigger malignancies remain largely unknown. Understanding these mechanisms would therefore contribute to the molecular basis for development of novel preventive, therapeutic and diagnostic approaches against cancer [3] . Chronic Hp infection of the gastric epithelium is strongly associated with the development of gastritis, peptic ulcers, mucosa-associated lymphoid tissue lymphoma and gastric cancer [4] , [5] . In gastric cancer, nearly 60% of all cases in developed countries and 75% in developing countries are attributed to chronic infection with Hp [6] . During persistent Hp colonization of the gastric mucosa, sustained inflammation and aberrant epithelial proliferation are considered to be major factors that lead to Hp-associated gastric diseases [5] , [7] , [8] , [9] , although the mechanisms underlying disease progression remain elusive. An accumulation of genetic and epigenetic alterations in normal tissues triggers carcinogenesis [9] , [11] . For example, DNA methylation of specific genes can be found in up to several percent of the cells in noncancerous gastric mucosae, and the rate of gene methylation is considered to be correlated with an increased risk of gastric cancer [10] , [11] , [12] , [13] . Importantly, Hp infection in the stomach has been shown to potentiate the induction of aberrant DNA methylation in the gastric epithelium, along with chronic inflammation [14] , [15] . Notably, methylation of promoter sites leads to gene expression silencing [14] , [15] . On the other hand, cumulative evidence suggests that microRNAs (miRNAs) might play important roles in the initiation and progression of various human diseases [16] , [17] . In this context, we sought to identify miRNAs that are causally involved in gastric malignancies associated with Hp infection by using several systematic and bioinformatic approaches and studying gastric epithelial cell lines, stomach tissue from Mongolian gerbils and human stomach biopsy specimens. In this comprehensive study, we demonstrate that miR-210 is a critical miRNA, which regulates gastric epithelial cell proliferation by targeting potential oncogenes. Furthermore, our work provides substantial evidence for the causal involvement of epigenetic silencing of miR-210 in development of gastric malignancies induced by chronic Hp infection. Accession codes: The microarray data have been deposited in Gene Expression Omnibus database under accession code GSE58004 . Epigenetic regulation of miRNAs during Hp infection Hp infection of the stomach has been shown to potentiate silencing of genes by aberrant DNA methylation in the gastric epithelium, due to chronic inflammation [14] , [15] . We hypothesized that chronic Hp infection could also lead to miRNA gene silencing by DNA methylation in gastric epithelia. To this end, we first examined miRNA expression levels in uninfected and Hp-infected gastric epithelial cells. Mongolian gerbils were infected intragastrically with 10 9 colony-forming unit (c.f.u.) Hp American Type Culture Collection (ATCC)43504 and gastric epithelial cells were examined for changes in miRNA expression levels 63 days after infection using a Taqman microRNA array. Several miRNAs, such as miR-210, miR-375 and miR-99a, were found to have reduced expression in the gastric epithelium of chronically Hp-infected gerbils, as compared with expression levels in uninfected gerbils ( Fig. 1a , Supplementary Figs 1a and 2 and Supplementary Data 1 ). 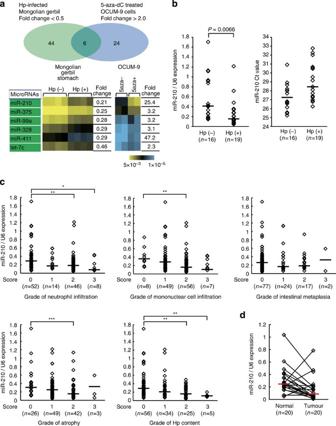Figure 1: miR-210 is downregulated during chronic Hp infection. (a) Mongolian gerbils were inoculated with Hp for 63 days. The gastric mucosae from uninfected (n=4) or infected (n=4) gerbils were subjected to a TaqMan-based miRNA microarray. OCUM-9 cells were treated with 1 μM 5-aza-dC for 4 days and subjected to a TaqMan-based miRNA microarray. The diagram represents the number of genes whose expression exhibited more than a twofold decrease in Hp-infected gerbils, as well as a more than twofold increase in 5-aza-dC-treated OCUM-9 cells. Gene numbers were obtained by examining gene lists generated by a twofold,P<0.001 criterions. Six genes overlapped with both groups were listed with a heat map. (b) The expression levels of miR-210 in human gastric mucosa were measured by real-time PCR. The horizontal bars indicate the mean value of each sample group. The Mann−WhitneyU-test was used to calculate theP-values. (c) The levels of miR-210 expression was assessed against degrees of neutrophil infiltration, mononuclear cell infiltration, intestinal metaplasia, atrophy and Hp content, according to the updated Sydney system20in 120 human gastric biopsy specimens. The miR-210 expression levels were measured by real-time PCR. The horizontal bars indicate the mean value of each sample group. *P<0.05, **P<0.01, ***P<0.001 by Mann–WhitneyU-test. (d) The levels of miR-210 of 20 paired gastric normal and tumor tissues. The miR-210 expression levels were measured by real-time PCR. The red horizontal bars indicate the mean value of each sample group. Figure 1: miR-210 is downregulated during chronic Hp infection. ( a ) Mongolian gerbils were inoculated with Hp for 63 days. The gastric mucosae from uninfected ( n =4) or infected ( n =4) gerbils were subjected to a TaqMan-based miRNA microarray. OCUM-9 cells were treated with 1 μM 5-aza-dC for 4 days and subjected to a TaqMan-based miRNA microarray. The diagram represents the number of genes whose expression exhibited more than a twofold decrease in Hp-infected gerbils, as well as a more than twofold increase in 5-aza-dC-treated OCUM-9 cells. Gene numbers were obtained by examining gene lists generated by a twofold, P <0.001 criterions. Six genes overlapped with both groups were listed with a heat map. ( b ) The expression levels of miR-210 in human gastric mucosa were measured by real-time PCR. The horizontal bars indicate the mean value of each sample group. The Mann−Whitney U -test was used to calculate the P -values. ( c ) The levels of miR-210 expression was assessed against degrees of neutrophil infiltration, mononuclear cell infiltration, intestinal metaplasia, atrophy and Hp content, according to the updated Sydney system [20] in 120 human gastric biopsy specimens. The miR-210 expression levels were measured by real-time PCR. The horizontal bars indicate the mean value of each sample group. * P <0.05, ** P <0.01, *** P <0.001 by Mann–Whitney U -test. ( d ) The levels of miR-210 of 20 paired gastric normal and tumor tissues. The miR-210 expression levels were measured by real-time PCR. The red horizontal bars indicate the mean value of each sample group. Full size image Although DNA methylation-mediated epigenetic silencing of miRNAs has previously been demonstrated [18] , the specific conditions of and mechanisms by which individual miRNA genes are silenced by methylation are not well described. To explore miRNA genes regulated by DNA methylation, we performed miRNA expression profiling in several samples of the OCUM-9 gastric cell line. A Taqman-based array analysis identified several genes, such as miR-411 and miR-210, with significantly increased expression in OCUM-9 cells treated with 5-aza-dC, a DNA methyltransferase inhibitor, suggesting that these miRNAs are probably silenced by DNA methylation in OCUM-9 cells ( Fig. 1a and Supplementary Fig. 1b ). We then reasoned that miRNAs which are both downregulated in Hp-infected gerbils and upregulated in 5-aza-dC-treated OCUM-9 cells are likely to be silenced by DNA methylation during chronic Hp infection. The genes that occur at the convergence of these two pools include miR-210, miR-375, miR-99a, miR-328, miR-411 and let-7c ( Fig. 1a ). Among them, we found miR-210 to be an intriguing candidate that might be regulated by epigenetic control during chronic Hp infection, as it appeared to be the most sensitive to DNA methylation (highly downregulated during chronic infection, and upregulated when methylation was inhibited). Together, the data presented here demonstrate that expression of several miRNA genes is epigenetically regulated by DNA methylation during chronic Hp infection. miR-210 is downregulated in Hp-infected gastric epithelium To examine the in vivo expression of miR-210 during the development of Hp-associated gastric illness, we further investigated epithelial cells in formalin-fixed, paraffin-embedded (FFPE) human gastric specimens from patients with or without Hp infection ( Supplementary Fig. 3 ). RNA samples from the gastric epithelia of FFPE specimens were examined for miR-210 expression using quantitative PCR with reverse transcription. The levels of miR-210 in Hp-positive gastric specimens were decreased compared with those in Hp-negative gastric specimens ( Fig. 1b ), consistent with a previous study of human gastric biopsy specimens [19] . To evaluate the clinical link between miR-210 downregulation and the progression of Hp-mediated gastritis, we collected 120 Hp-positive human gastric specimens and characterized the severity of gastritis according to the Sydney system [20] ( Fig. 1c ). We found that the levels of miR-210 expression decreased in parallel with increased grades of neutrophil infiltration, mononuclear cell infiltration, atrophy and Hp content ( Fig. 1c ). In addition, we assessed miR-210 expression in distinct normal and tumour areas in biopsies from 20 gastric cancer patients, and found significantly higher miR-210 levels in normal regions as compared within tumour regions ( Fig. 1d ). As reported previously [21] , [22] , some cancerous regions displayed higher miR-210 levels than did normal regions. As miR-210 is known to be upregulated in hypoxic conditions, this is perhaps due to the occurrence of local hypoxia inside solid tumours [21] . We could therefore surmise that miR-210 expression is suppressed concurrently with the progression of Hp-mediated gastric lesions. A CpG island in miR-210 is methylated in Hp-infected stomach Given the downregulation of miR-210 in Hp-mediated gastric lesions, we sought to examine the possible regulation of miR-210 by DNA methylation during chronic Hp infection. The miR-210 genomic locus contains a CpG island that overlaps with the miR-210 -coding sequence and extends upstream into the miR-210 promoter region ( Fig. 2a ). To test if the methylation status of this CpG island changes during chronic Hp infection, we examined the stomach FFPE specimens obtained from Hp-positive or Hp-negative adults, to assess the extent of CpG methylation within miR-210 by bisulphite sequencing. We measured two distinct regions, named bisulphite sequencing 1 and bisulphite sequencing 2, within the CpG island ( Fig. 2a,b ). Region 1 was found to have a higher degree (50.3%) of methylation in Hp-positive stomach tissue than in Hp-negative stomachs (31.1%) ( Fig. 2b ). Analysis of the second region displayed a similar trend in methylation status (40.9% in Hp-positive and 13.6% in Hp-negative tissues) ( Fig. 2b ). In addition, we analysed four distinct regions by methylation-specific PCR (MSP), and all four, MSP1, MSP2, MSP3 and MSP4, were found to be more methylated in Hp-positive stomach specimens than in Hp-negative stomachs ( Fig. 2a,c ). Together our analyses strongly pointed to a significantly higher rate of CpG methylation within the miR-210 locus in Hp-positive versus Hp-negative individuals. Increased miR-210 methylation was also observed in human inflammatory bowel disease specimens ( Supplementary Fig. 4 ), indicating that a persistent inflammatory process is probably important for the induction of DNA methylation. 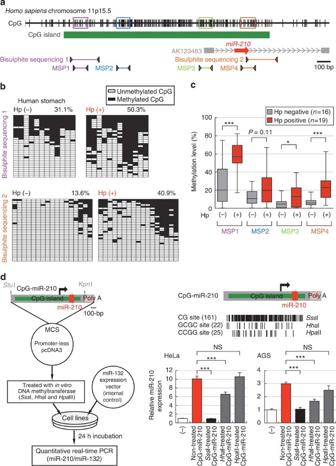Figure 2: miR-210 expression is epigenetically silenced during chronic Hp infection. (a) A schematic diagram of the CpG island and CpG sites in the miR-210 locus on human chromosome 11p15.5. miR-210 and the transcription start site of pri-miR-210 are in the CpG island. The green bar, CpG island; open rectangles, methylation-specific PCR (MSP) regions; closed arrowheads and bars (purple, blue, green or orange), bisulphite sequenced and MSP regions. (b) Bisulphite sequencing of the miR-210 CpG island in human gastric biopsy samples. Each box indicates the methylation status of the CpG site. Over 40 clones from each mixed sample were sequenced. Each row represents an individual sequenced DNA strand. The percent methylation in each sequenced region was indicated. (c) MSP analysis on the DNA methylation levels of miR-210 in human gastric mucosa biopsies. The ratios were calculated by the number of methylated CGs versus the number of methylated and unmethylated CGs. All plots show the 25th–75th percentiles (boxes) and 5th–95th percentiles (whiskers). The line in each box represents the median. *P<0.05, **P<0.01, ***P<0.001 by Mann–WhitneyU-test. (d) A schematic representation of the assay system for DNA methylation-dependent regulation of miR-210 expression. The CpG-miR-210 plasmid contains themiR-210CpG island and an artificially added poly-A site within the multicloning site (MCS) of promoter-less pcDNA3 plasmid. The CpG island sequence was derived from human chromosome 11: 557,848−559,554 (NCBI36/hg18). The black vertical bars indicate the CpG methylation sites recognizedin vitroby each DNA methyltransferase. The CpG-miR-210 expression vector was treatedin vitrowith each DNA methyltransferase ofSssI (CG to mCG),HhaI (GCGC to GmCGC) andHpaII (CCGG to CmCGG). Each DNA was transfected into HeLa or AGS cells together with a cytomegalovirus (CMV)-derived miR-132 expression vector (internal control). The relative expression of miR-210/miR-132 was quantified by real-time PCR. The error bars indicate s.d. (n=3). *P<0.05, **P<0.01, ***P<0.001, NS (not significant) by Student’st-test. Figure 2: miR-210 expression is epigenetically silenced during chronic Hp infection. ( a ) A schematic diagram of the CpG island and CpG sites in the miR-210 locus on human chromosome 11p15.5. miR-210 and the transcription start site of pri-miR-210 are in the CpG island. The green bar, CpG island; open rectangles, methylation-specific PCR (MSP) regions; closed arrowheads and bars (purple, blue, green or orange), bisulphite sequenced and MSP regions. ( b ) Bisulphite sequencing of the miR-210 CpG island in human gastric biopsy samples. Each box indicates the methylation status of the CpG site. Over 40 clones from each mixed sample were sequenced. Each row represents an individual sequenced DNA strand. The percent methylation in each sequenced region was indicated. ( c ) MSP analysis on the DNA methylation levels of miR-210 in human gastric mucosa biopsies. The ratios were calculated by the number of methylated CGs versus the number of methylated and unmethylated CGs. All plots show the 25th–75th percentiles (boxes) and 5th–95th percentiles (whiskers). The line in each box represents the median. * P <0.05, ** P <0.01, *** P <0.001 by Mann–Whitney U -test. ( d ) A schematic representation of the assay system for DNA methylation-dependent regulation of miR-210 expression. The CpG-miR-210 plasmid contains the miR-210 CpG island and an artificially added poly-A site within the multicloning site (MCS) of promoter-less pcDNA3 plasmid. The CpG island sequence was derived from human chromosome 11: 557,848−559,554 (NCBI36/hg18). The black vertical bars indicate the CpG methylation sites recognized in vitro by each DNA methyltransferase. The CpG-miR-210 expression vector was treated in vitro with each DNA methyltransferase of Sss I (CG to mCG), Hha I (GCGC to GmCGC) and Hpa II (CCGG to CmCGG). Each DNA was transfected into HeLa or AGS cells together with a cytomegalovirus (CMV)-derived miR-132 expression vector (internal control). The relative expression of miR-210/miR-132 was quantified by real-time PCR. The error bars indicate s.d. ( n =3). * P <0.05, ** P <0.01, *** P <0.001, NS (not significant) by Student’s t -test. Full size image To elucidate the causal link between miR-210 downregulation and higher DNA methylation at the CpG island of the miR-210 locus, we cloned the sequence encompassing miR-210 and part of the CpG island onto a plasmid vector, to further investigate the effect of DNA methylation on miR-210 expression in vitro ( Fig. 2d ). The miR-210-containing vectors were treated with DNA methyltransferases Sss I, Hha I or Hpa II before transfection into epithelial cells. When the CpG island-containing miR-210 was completely methylated using Sss I (CG→mCG), miR-210 expression levels were markedly reduced in epithelial cells ( Fig. 2d ). On the other hand, a partially methylated CpG-miR-210, resulting from Hha I or Hpa II treatment (GCGC→CmCGG), had a moderate-to-none effect on miR-210 expression ( Fig. 2d ), strongly suggesting that miR-210 expression can be influenced by the methylation status of several CpG sites in a site-specific and dose-dependent manner. Additionally, there was a modest inverse correlation between the miR-210 expression levels and the methylation levels of the CpG island around the miR-210-coding region in various gastric epithelial cell lines, including MKN7, AGS, MKN1, OCUM-8, SH-10-Tc, NCI-N87, OCUM-1, OCUM-2D, MKN74, MKKN45, OCUM-2M, AZ521, OCUM-12 and OCUM-9 ( Supplementary Fig. 5 ). Altogether, we conclude that the level of DNA methylation occurring within the CpG island affects miR-210 expression, and that reduced miR-210 expression in Hp-infected stomach tissue results, at least in part, from DNA methylation of the miR-210 CpG island. miR-210 activity suppresses gastric cell proliferation To pursue the biological impact of deregulated miR-210 expression on the gastric epithelium during Hp infection, we introduced double-stranded miR-210 into various gastric epithelial cell lines, including MKN45, AGS, OCUM-9 and OCUM-2D, and investigated the effect of high levels of miR-210 expression on epithelial cell proliferation. Cell viability was significantly decreased by miR-210 overexpression after 96 h of incubation ( Fig. 3a and Supplementary Fig. 6a ). In contrast, there was a modest increase in proliferation of AGS and OCUM-2D cells transfected with the miR-210 inhibitor anti-miR-210 for 96 h, as compared with control cells transfected with anti-miR-Nega ( Fig. 3b ). Levels of miR-210 were reduced by approximately 30% in anti-miR-210-overexpressing AGS cells, measured by real-time PCR analysis ( Supplementary Fig. 6a ). To confirm the specific action of miR-210, we studied the effects of miR-210 overexpression in MKN45 cells by transfecting miR-210 or miR-210 mut (mutations introduced into the seed sequence [23] , required for target gene recognition). Relative miR-210 expression levels and viable cells were measured after 96 h of transfection ( Fig. 3c and Supplementary Fig. 6b ). Cells overexpressing miR-210 but not miR-210 mut displayed decreased viability in a dose-dependent manner ( Fig. 3c ). To verify the effects of miR-210 on the cell cycle, we transfected miR-210, miR-210 mut or miR-Nega control into MKN45 cells. Two days post transfection, cells were stained with propidium iodide and analysed by flow cytometry to visualize nuclei and thereby assess cell cycle progression. Cells overexpressing miR-210 but not the negative control or the miR-210 mut construct were found largely to be in the G1 phase, and less so in G2/M and S phases ( Fig. 3d ). Together, these results strongly suggest that reduced miR-210 expression might lead to cell cycle induction, dependent on a functional seed sequence. 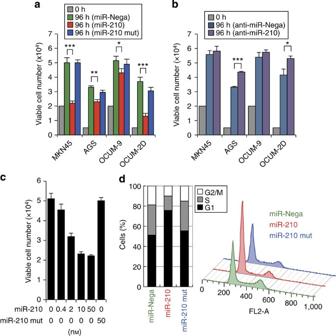Figure 3: miR-210 regulates gastric cell proliferation. (a) The indicated gastric cells were transfected with 50 nM of miR-210 or miR-210 mut (mutant) and assessed for cell viability 4 days later. The data indicate average values calculated from triplicates. Error bars show s.d. (n=3). (b) The gastric cell lines were transfected with 50 nM of anti-miR-Nega or anti-miR-210 and assessed for cell viability 4 days later. The data shown are average values calculated from triplicates. Error bars show s.d. (n=3). (c) MKN45 cells were transfected with the indicated concentration of miR-210 or mutant miR-210 and assessed for cell viability 4 days later. The error bars indicate s.d. (n=3). (d) MKN45 cells were transfected with an miRNA-negative control, miR-210 or a mutant miR-210. After 2 days, the cells were stained with propidium iodide and analysed by flow cytometry. *P<0.05, **P<0.01, ***P<0.001, NS, not significant by Student’st-test. Figure 3: miR-210 regulates gastric cell proliferation. ( a ) The indicated gastric cells were transfected with 50 nM of miR-210 or miR-210 mut (mutant) and assessed for cell viability 4 days later. The data indicate average values calculated from triplicates. Error bars show s.d. ( n =3). ( b ) The gastric cell lines were transfected with 50 nM of anti-miR-Nega or anti-miR-210 and assessed for cell viability 4 days later. The data shown are average values calculated from triplicates. Error bars show s.d. ( n =3). ( c ) MKN45 cells were transfected with the indicated concentration of miR-210 or mutant miR-210 and assessed for cell viability 4 days later. The error bars indicate s.d. ( n =3). ( d ) MKN45 cells were transfected with an miRNA-negative control, miR-210 or a mutant miR-210. After 2 days, the cells were stained with propidium iodide and analysed by flow cytometry. * P <0.05, ** P <0.01, *** P <0.001, NS, not significant by Student’s t -test. Full size image Identification of miR-210 target genes in gastric cells miRNAs bind to the 3′ untranslated region (UTR) of target gene mRNAs and enhance their degradation [24] . We screened for miR-210 target genes in gastric epithelial cells by performing a cDNA microarray and bioinformatics analysis ( Fig. 4a ). We overexpressed miR-210 by introducing 50 nM pre-miR-210 into MKN45 or AGS cells and collected total RNA 36 h after transfection. We screened a total of 20,886 genes using a cDNA microarray, and found 146 and 237 genes in MKN45 and AGS cells, respectively, that were downregulated at least 60% in the presence of miR-210 as compared with miR-Nega. ( Fig. 4a , Supplementary Tables 1 and 2 , and Supplementary Fig. 7 ). Using TargetScan ver. 6.2 ( http://www.targetscan.org/ ), we were able to identify genes containing a putative miR-210 seed sequence in the 3′UTR. There are three characteristics of miR-210 seed sequences called 8-mer, 7mer-m8 and 7mer-A1 (ref. 23) [23] . These categories have hierarchy of site efficacy: 8-mer>7mer-m8>7mer-A1. Of the 28 genes suppressed by miR-210 in both MKN45 and AGS cells, 12 genes possessed a miR-210 target sequence ( Fig. 4a and Supplementary Table 3 ). 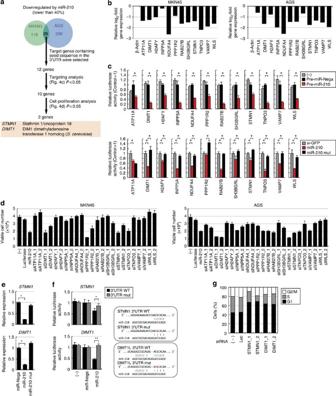Figure 4: miR-210 regulates gastric cell proliferation by targetingSTMN1andDIMT1. (a) A schematic diagram of the strategy used to identify miR-210 target genes involved in gastric cell proliferation. (b) The expression levels of 12 genes in MKN45 or AGS cells transfected with pre-miR-210 were measured by real-time PCR. The fold change of each gene was calculated by normalizing to the gene expression level of cells transfected with the pre-miRNA-negative control. All genes were significantly downregulated by pre-miR-210 (n=3,P<0.05 by Student’st-test). (c) The 3'UTR sequence of each gene was cloned downstream of the luciferase reporter vector. Each reporter plasmid and the small RNAs indicated in the figure were transfected into 293T cells, and luciferase assays were performed. The levels of luciferase activity in 293T cells overexpressing pre-miR-210 or miR-210 were compared with each control of pre-miR-Nega or miR-210 mut (mutant), respectively, by Student’st-test. Error bars show s.d. (n=4). *P<0.05 by Student’st-test. (d) MKN45 or AGS cells were transfected with the indicated siRNAs, and cell viability was measured 4 days later. Two independent siRNAs were used for each gene. Error bars show s.d. (n=3). (e) The relative mRNA levels ofSTMN1andDIMT1in miR-210, miR-210 mut, or miR-Nega-transfected AGS cells are shown. The data indicate the means±s.d. (n=3). *P<0.001 by Student’st-test. (f) Left panel; luciferase vectors containing the 3'UTR (3'UTR WT) of each gene and mutant vectors possessing mutated target sites (3' UTR mut) were constructed. The reporter vectors and miR-210 were co-transfected into 293T cells and subjected to luciferase assays. The means±s.d. (n=4) are shown. Right panel; part of the luciferase vector sequences for theSTMN1andDIMT13'UTRs. The sequences in red characters are the mutated miR-210 target sites. *P<0.05, **P<0.001 by Student’st-test. (g)STMN1andDIMT1regulate the cell cycle of MKN45 cells. MKN45 cells were transfected with the indicated siRNAs at a final concentration of 50 nM. The cell cycle phase was analysed using propidium iodide staining and flow cytometry. Two independent siRNAs were used for each gene. Figure 4: miR-210 regulates gastric cell proliferation by targeting STMN1 and DIMT1. ( a ) A schematic diagram of the strategy used to identify miR-210 target genes involved in gastric cell proliferation. ( b ) The expression levels of 12 genes in MKN45 or AGS cells transfected with pre-miR-210 were measured by real-time PCR. The fold change of each gene was calculated by normalizing to the gene expression level of cells transfected with the pre-miRNA-negative control. All genes were significantly downregulated by pre-miR-210 ( n =3, P <0.05 by Student’s t -test). ( c ) The 3'UTR sequence of each gene was cloned downstream of the luciferase reporter vector. Each reporter plasmid and the small RNAs indicated in the figure were transfected into 293T cells, and luciferase assays were performed. The levels of luciferase activity in 293T cells overexpressing pre-miR-210 or miR-210 were compared with each control of pre-miR-Nega or miR-210 mut (mutant), respectively, by Student’s t -test. Error bars show s.d. ( n =4). * P <0.05 by Student’s t -test. ( d ) MKN45 or AGS cells were transfected with the indicated siRNAs, and cell viability was measured 4 days later. Two independent siRNAs were used for each gene. Error bars show s.d. ( n =3). ( e ) The relative mRNA levels of STMN1 and DIMT1 in miR-210, miR-210 mut, or miR-Nega-transfected AGS cells are shown. The data indicate the means±s.d. ( n =3). * P <0.001 by Student’s t -test. ( f ) Left panel; luciferase vectors containing the 3'UTR (3'UTR WT) of each gene and mutant vectors possessing mutated target sites (3' UTR mut) were constructed. The reporter vectors and miR-210 were co-transfected into 293T cells and subjected to luciferase assays. The means±s.d. ( n =4) are shown. Right panel; part of the luciferase vector sequences for the STMN1 and DIMT1 3'UTRs. The sequences in red characters are the mutated miR-210 target sites. * P <0.05, ** P <0.001 by Student’s t -test. ( g ) STMN1 and DIMT1 regulate the cell cycle of MKN45 cells. MKN45 cells were transfected with the indicated siRNAs at a final concentration of 50 nM. The cell cycle phase was analysed using propidium iodide staining and flow cytometry. Two independent siRNAs were used for each gene. Full size image We examined these 12 genes using real-time PCR and found that all 12 genes, ATP11A, DIMT1, H2AFY, INPP5A, NDUFA4, PPP1R2, RAB27B, SH3BGRL, STMN1, TNPO3, VAMP7 and WLS , were strongly suppressed by miR-210 in both MKN45 and AGS cells ( Fig. 4a,b , and Supplementary Table 3 ). Importantly, 11 out of the 12 genes possessed either 7mer-m8 or the 8-mer seed sequence in their 3′UTR sequence ( Supplementary Fig. 8 ). We subsequently asked whether the suppression of these 12 genes by miR-210 was mediated by 3′UTR targeting ( Fig. 4c ). To this end, the 3′UTR sequences of the 12 miR-210 targeted genes were fused with the firefly luciferase gene in a reporter plasmid and luciferase activity was measured in 293T cells exogenously co-expressing miR-210 for 36 h. The results suggested that all genes except for ATP11A and PPP1R2 can be suppressed by miR-210 expression ( Fig. 4c ). STMN1 and DIMT1 modulate gastric cell proliferation We subsequently screened these 12 genes for effects on gastric epithelial cell proliferation by siRNA against each miR-210 target ( Fig. 4d , Supplementary Fig. 9 and Supplementary Table 4 ). Four days post transfection with 50 nM of each siRNA, we measured the extent of cell proliferation in MKN45 and AGS cells. Inhibition of some genes, especially STMN1 (also termed stathmin1, oncoprotein 18 or metablastin) and DIMT1 (also termed DIM1, demethyladenosine transferease 1), showed a decrease in cell proliferation in both cell lines ( Fig. 4a,d ). STMN1 is a well-known protein upregulated in solid tumours, and is involved in the initiation of tumour development [25] , [26] , [27] , [28] . However, the biological functions of DIMT1, which belongs to the S -adenosylmethionine-dependent methyltransferase superfamily, are unknown in cancer. Thus, having experimentally identified 10 genes as novel miR-210 targets in this study, we determined that at least two, STMN1 and DIMT1 , may play specific roles in tumorigenesis. We sought to further characterize the biological role of STMN1 and DIMT1 as miR-210 target genes, and first studied the effect of miR-210 overexpression on target gene expression. AGS cells transfected with miR-210 or miR-210 mut were assessed for STMN1 and DIMT1 gene expression. Expression of miR-210 but not miR-210 mut led to suppressed levels of STMN1 and DIMT1 ( Fig. 4e ). We also created a series of luciferase reporter plasmids encoding wild type (WT) and mutated forms of the 3′UTR of STMN1 or DIMT1 ( Fig. 4f ). Each of the reporter plasmids were co-transfected with miR-210 vectors into 293T cells, and luciferase activity was measured 36 h post transfection. Expression levels of STMN1 and DIMT1 with WT 3′UTR regions were dampened in the presence of miR-210, but the 3′UTR mutants were not ( Fig. 4f ), implying that miR-210 regulation of STMN1 and DIMT1 gene expression occurs via their 3′UTR seed sequences. Indeed, this notion was further supported by a bioinformatics approach using mRNA target prediction programs provided by TargetScan, miRanda, Diana Micro-T and PITA ( Supplementary Fig. 10a ). Furthermore, overexpression of STMN1 or DIMT1 in MKN45 cells led to increased cell proliferation as compared with control cells ( Supplementary Fig. 10b ). Lastly, we investigated whether siRNA expression against each of the miR-210 target genes would lead to cell cycle arrest. We detected an accumulation of cells in the G1 phase when MKN45 cells were treated with siRNA against target genes for 2 days ( Fig. 4g and Supplementary Fig. 10c ). Based on these results, we conclude that miR-210 modulation of STMN1 and DIMT1 gene expression may be the mechanism by which chronic Hp infection promotes proliferation of gastric epithelial cells. STMN1 and DIMT1 are highly expressed in Hp-infected stomach To test the hypothesis that miR-210 regulates cell proliferation through STMN1 and DIMT1 in the stomachs of patients suffering from Hp chronic infection, we examined the mRNA expression levels of these three genes in FFPE Hp-positive and Hp-negative gastric human sections using PCR with reverse transcription. mRNA levels of both STMN1 and DIMT1 were upregulated in Hp-positive stomachs ( n =19) as compared with Hp-negative control stomachs ( n =16) ( Fig. 5 ). To confirm this, we employed our Mongolian gerbil stomach model to investigate miRNA expression levels in gastric epithelial cells. Gerbils were infected intragastrically with 10 9 c.f.u. of Hp ATCC43504, miR-210 expression levels were measured 63 days post infection. miR-210 expression was found to be lower in Hp-infected gerbil stomachs as compared with uninfected stomachs ( Fig. 6a,b ). In contrast to WT infection, we found that gerbils infected with a cagA deletion mutant strain (Δ cagA ) of ATCC43504 showed no decrease in miR-210 expression in the stomach, as compared with uninfected stomachs ( Fig. 6a and Supplementary Fig. 11a ), CagA is a major pathogenic factor for Hp-induced inflammation [29] , [30] , and our results suggest that CagA also plays an important role in suppression of miR-210. Moreover, expression of Stmn1 and Dimt1 was much higher in the gastric tissue of Hp-infected gerbil stomachs, whereas miR-210 was barely detected in the lamina propria ( Fig. 6a–c , and Supplementary Fig. 11b ). Importantly, PCNA (proliferating cell nuclear antigen)-positive epithelial cells were significantly more abundant in Hp-positive gastric tissue than in Hp-negative gastric tissue ( Fig. 6d ). Furthermore, STMN1 and PCNA protein levels were increased in the gastric mucosa of Hp-infected gerbils as compared with uninfected gerbils ( Supplementary Fig. 11c ). Taken together, we can conclude that miR-210 plays a key role in regulating proliferation of gastric epithelial cells, by targeting a set of genes including STMN1 and DIMT1 . 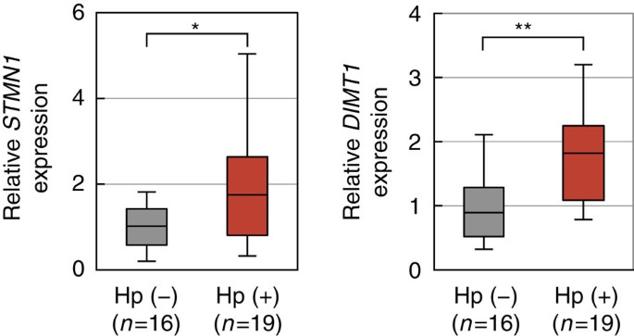Figure 5: Expression levels ofSTMN1andDIMT1are increased in gastric biopsy samples from Hp-infected individuals. mRNA expression levels were quantified by real-time PCR. All plots show the 25th–75th percentiles (boxes) and 5th–95th percentiles (whiskers). The line in each box represents the median. *P<0.05, **P<0.01 by Mann−WhitneyU-test. Figure 5: Expression levels of STMN1 and DIMT1 are increased in gastric biopsy samples from Hp-infected individuals. mRNA expression levels were quantified by real-time PCR. All plots show the 25th–75th percentiles (boxes) and 5th–95th percentiles (whiskers). The line in each box represents the median. * P <0.05, ** P <0.01 by Mann−Whitney U -test. 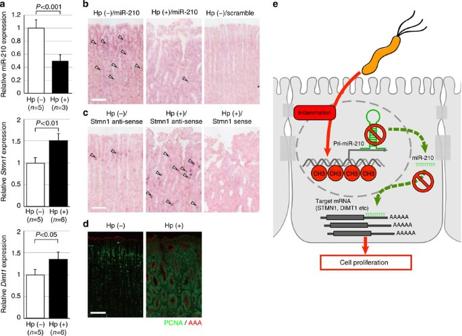Figure 6: Decreased miR-210 expression is associated with increased levels ofStmn1and proliferation-related marker in Hp-infected Mongolian gerbils. (a) Mongolian gerbils were inoculated with Hp, and 63 days later, gastric mucosa tissues were isolated from uninfected (Hp (−),n=5) and infected (Hp (+),n=3 for miR-210 andn=6 for mRNA) gerbils. The expression levels of miR-210,Stmn1andDimt1were quantified by real-time PCR analysis. The Mann−WhitneyU-test was used to calculateP-values. (b) Detection of miR-210 in the gastric sections from Hp-infected Mongolian gerbils byin situhybridization. Gastric sections from uninfected (Hp (−)) or infected (Hp (+)) were stained with the indicated probes, and counterstained with Kernechtrot stain. The scramble probe was used for background staining. Scale bar, 100 μm. (c)In situhybridization ofStmn1in the stomach sections from Hp-infected animals. The sense probe was used for background staining. Scale bar, 100 μm. (d) Nine weeks after infection, the gerbils were killed, and stomach sections were immunostained with PCNA (proliferating cells, green) and AAA (pit cells, red). Scale bar, 100 μm. (e) Gene silencing of miR-210 upregulates target gene expression and promotes aberrant gastric epithelial cell proliferation during chronic Hp infection. Full size image Figure 6: Decreased miR-210 expression is associated with increased levels of Stmn1 and proliferation-related marker in Hp-infected Mongolian gerbils. ( a ) Mongolian gerbils were inoculated with Hp, and 63 days later, gastric mucosa tissues were isolated from uninfected (Hp (−), n =5) and infected (Hp (+), n =3 for miR-210 and n =6 for mRNA) gerbils. The expression levels of miR-210, Stmn1 and Dimt1 were quantified by real-time PCR analysis. The Mann−Whitney U -test was used to calculate P -values. ( b ) Detection of miR-210 in the gastric sections from Hp-infected Mongolian gerbils by in situ hybridization. Gastric sections from uninfected (Hp (−)) or infected (Hp (+)) were stained with the indicated probes, and counterstained with Kernechtrot stain. The scramble probe was used for background staining. Scale bar, 100 μm. ( c ) In situ hybridization of Stmn1 in the stomach sections from Hp-infected animals. The sense probe was used for background staining. Scale bar, 100 μm. ( d ) Nine weeks after infection, the gerbils were killed, and stomach sections were immunostained with PCNA (proliferating cells, green) and AAA (pit cells, red). Scale bar, 100 μm. ( e ) Gene silencing of miR-210 upregulates target gene expression and promotes aberrant gastric epithelial cell proliferation during chronic Hp infection. Full size image Our current study identified downregulation of miR-210 as a risk factor for development of Hp-associated gastric diseases including cancer. Furthermore, we have provided substantial evidence supporting the causal link between suppression of miR-210 expression and epigenetic modification of the DNA sequence encompassing the miR-210 gene, highlighting DNA methylation as a mechanism for epigenetic silencing of miRNA genes during chronic inflammation. Since aberrant DNA methylation has also been reported in other chronic inflammatory diseases, including ulcerative colitis and hepatitis virus B-associated chronic hepatitis [11] , [12] , [13] , [31] , [32] , that are causative for cancers, we predict that similar inflammation-induced DNA methylation leading to miRNA gene silencing could be an underlying tumorigenic mechanism associated with those diseases. Therefore, it will be of particular interest to identify miRNA genes sensitive to pathogenic DNA methylation, as well as the affected miRNA target genes in specific disease states. In addition, the molecular mechanisms of how chronic inflammation causes an increase in DNA methylation is an important question to pursue in future studies. There is some discrepancy concerning the status of miR-210 as a carcinogenic miRNA. Some studies find augmented miR-210 expression in solid tumours [21] , [22] , [33] , [34] , while others see reduced expression in ovarian cancer [35] . In our study, miR-210 levels were lower in Hp-positive human stomachs than in Hp-negative human stomachs ( Fig. 1b ). Moreover, miR-210 expression was variable even within the stomachs of gastric cancer patients; tumour areas displayed significantly lower miR-210 expression than tissue biopsies from normal areas ( Fig. 1d ). The varying levels of miR-210 found in different solid tumours could be explained in part by the different states of hypoxia present during distinct stages of cancer. After enhanced formation of a solid tumour, a low-oxygen state might be dominant, leading to higher levels of miR-210 [21] , [33] , [34] . As robust methylation is induced by prolonged inflammation [36] , miR-210 expression levels might be affected by an altered balance of hypoxia and inflammation in distinct cancer states. Our data show that miR-210 levels are reduced in Hp-positive gastric specimens, while the miR-210-associated CpG island is hypermethylated ( Fig. 2b,c ). This suggests that sustained downregulation of miR-210 by CpG island methylation could cause prolonged aberrant proliferation of gastric epithelial cells during chronic Hp infection, thus supporting a micro-tumorigenic environment. Although previous studies have reported an association between inflammatory diseases and aberrant expression of miRNAs, some of which have been also shown to be DNA methylated [37] , [38] , [39] , few groups have demonstrated in vivo evidence for the causal link between affected miRNAs and their targets during disease progression. Our comprehensive analysis identified 12 genes that are downregulated in response to miR-210 overexpression ( Fig. 4a and Supplementary Table 3 ), most of which had not been previously characterized as miR-210 targets. The siRNA inhibition experiments described in this study suggest that the activities of STMN1 and DIMT1 regulate gastric epithelial proliferation more profoundly than other genes ( Fig. 4d ). STMN1 has been characterized as an oncoprotein (also known as oncoprotein 18), associated with gastric and other various types of cancer [26] , [27] , [28] . Therefore, our discovery of STMN1 upregulation in Hp-positive stomachs, where miR-210 levels are very low, suggests that it is an important factor in the development of gastric cancer on chronic Hp infection. Given that the increase in DNA methylation of the miR-210 gene, is correlated with disease progression ( Fig. 1c ), we propose a novel pathophysiological pathway promoting aberrant gastric epithelial cell proliferation on chronic infection by Hp ( Fig. 6e ). In conclusion, our results demonstrate that epigenetic silencing of miR-210 following Hp infection enhances the proliferation of gastric epithelial cells. Our findings should therefore help to further understand how chronic Hp infection of the gastric mucosa becomes a risk for gastric cancer, and to identify targets for future research which will be aimed at developing new drugs and markers for tumour differentiation. Human biopsy samples and Hp infection of Mongolian gerbils Primary gastric mucosa samples from 35 patient volunteers were obtained to investigate miR-210, STMN1 , DIMT1 , U6 and ACTB expression and to analyse DNA methylation levels in Hp-infected gastric tissue. The study included 19 Hp-positive cases and 16 Hp-negative cases. Due to ethical considerations, we were unable to test with tissues from healthy volunteers. An additional 85 primary gastric mucosa samples were obtained to measure the levels of miR-210 and U6. These samples were scored depending on the severity of neutrophil infiltration, mononuclear cell infiltration, intestinal metaplasia, atrophy and Hp content, according to the updated Sydney system [20] . These samples were acquired from the archives of the Department of Pathology at the University of Tokyo Hospital. Hp infection was diagnosed in the biopsies by haematoxylin and eosin staining and confirmed by real-time PCR analysis of Hp rRNA from total RNA. The 20 gastric tumour samples and paired gastric normal tissues were obtained to analyse miR-210 and U6 expression levels. Tissues were fixed in neutral-buffered formalin and embedded in paraffin blocks for RNA extraction. FFPE were sectioned to a 10-μm thickness for RNA or DNA extraction. Total RNA, including miRNA, or total DNA was extracted from the paraffin-embedded tissues of surgically resected samples with a RecoverAll Total Nucleic Acid Isolation Kit for FFPE Tissues (Ambion). Informed consent was obtained from all human subjects involved, and all aspects of this study were approved by the University of Tokyo Ethics Committee. For the in vivo infection model, 6-week-old male MGS/Sea Mongolian gerbils ( Meriones unguiculatus ; CLEA Japan) were intragastrically inoculated with a bacterial culture containing 10 9 c.f.u. of Hp (ATCC43504) in Brucella broth containing 5% (v/v) fetal calf serum. Control animals were orally administered Brucella broth containing only 5% (v/v) fetal calf serum. To isolate RNA, the gastric mucosal tissues were immediately harvested and frozen in liquid nitrogen. Total RNA was extracted using ISOGEN (Nippon gene) after the stomach tissue was homogenized. All animal experiments were conducted in accordance with the guidelines of the University of Tokyo for the care and use of laboratory animals and were approved by the ethics committee for animal experiments of the University of Tokyo. cDNA microarray analysis AGS or MKN45 cells were transfected with 50 nM of pre-miRNA-negative control #1 (miR-Nega) (Life technologies, Ambion) or pre-miRNA miR-210 for 36 h using Lipofectamine RNAiMAX (Invitrogen). Total RNA was purified using an RNeasy Kit (Qiagen) according to the manufacturer’s instructions. Gene expression profiling was performed using the Affymetrix Human Genome U133A Plus 2.0 Array (Affymetrix), to analyse over 47,000 transcripts, including ~21,000 well-characterized human genes, according to the manufacturer’s instructions. The data were normalized and analysed by GeneSpring GX 7.3 (Agilent Technologies). Target genes containing miR-210 seed sequences were identified by Human TargetScan 6.2 ( http://www.targetscan.org/ ). Genes with expression levels lower than 40% of the miR-Nega-transfected control cells, after miR-210 overexpression, and containing miR-210 target sites in their 3'UTRs, were considered to be candidates for miR-210 targeting. mRNA array Mongolian gerbils were inoculated with a bacterial culture containing 10 9 c.f.u. of Hp (ATCC43504), and total RNA containing the small RNA fraction was purified from gastric tissues at 63 days post infection using the miRNeasy Mini Kit (Qiagen), according to the manufacturer’s instructions. OCUM-9 cells were treated with 1 μM 5-aza-dC for 4 days. Total RNA was purified as described above. The total RNA was reverse transcribed for 1st strand synthesis using PCRMegaplex Primer Pool RT primers (Applied Biosystems). The miRNA expression profile of OCUM-9 cells or control cells was determined using Human TaqMan Array MicroRNA Cards A (Applied Biosystems). The miRNA expression profile of Mongolian gerbils was determined using Rodent TaqMan Array MicroRNA Cards (Applied Biosystems). PCR reactions were performed using TaqMan Universal PCR Master Mix No AmpErase UNG (2 × ) with a 7900HT thermocycler (Applied Biosystems) and the manufacturer’s recommended programme. The expression profile for each miRNA was analysed using the ΔΔCt method and the expression levels were calculated using U6 expression as an internal control. For the miRNA array with OCUM-9 cells, SNU48 was used as an internal control. Heat maps were produced with Java TreeView software ( http://jtreeview.sourceforge.net/ ). Cell cycle analysis and cell proliferation assay For cell cycle analysis, MKN45 cells were fixed in 70% ethanol overnight at −20 °C. After washing with phosphate-buffered saline (PBS), the cells were incubated with 10 mg ml −1 RNase A (Sigma) and 50 μg ml −1 propidium iodide in PBS for 2 h on ice in the dark. Cell cycle data were collected with a FACSCalibur flow cytometer (BD Biosciences immunocytochemistry system) and analysed with CellQuest and FlowJo software. For the cell proliferation assay, transiently transfected AGS and MKN45 cells were cultured in RPMI-1640 (Invitrogen) containing 10% fetal bovine serum, and OCUM-9 or OCUM-2D cells were cultured in Dulbecco’s modified eagles medium containing 10% fetal bovine serum, 2 mM glutamine and 0.5 mM sodium pyruvate. After the indicated time period, the culture medium was replaced with medium containing 10 μl per well of the substrate for the Cell Counting Kit-8 (Dojindo Laboratories). Briefly, the plates were shaken for 10 s and incubated at 37 °C for 1 h. Then, the absorbance at 450 nm for each well was measured using a Varioskan Flash (Thermo Scientific). The morphological changes of each cell were observed using an Axiovert 135-SENSYS (Carl Zeiss MicroImaging). Quantitative real-time PCR To measure gene expression levels, including pri-miR-210, total RNA was reverse transcribed into cDNA with oligo (dT) primers and random hexamer primers using ReverTra Ace (TOYOBO Life Science). Real-time PCR was performed using a LightCycler DX400 (Roche) and SYBR Premix Ex Taq II (TaKaRa) according to the manufacturers’ protocols. Relative mRNA expression was calculated using the human β-actin gene as an endogenous reference standard. The specificity of the PCR products was confirmed by melting-curve analysis. To determine the mature miR-210 expression levels, total RNA was isolated from cell lines using an miRNeasy Mini Kit (Qiagen). Total RNA was used in reverse transcriptase and subsequent pre-amplification reactions using the miScript Reverse Transcription Kit and the manufacturer’s protocol (Qiagen). miRNA real-time PCR was performed to detect miRNAs and U6 using a miScript SYBR Green PCR Kit (Qiagen). The specificity of the PCR products was confirmed by melting-curve analysis. The miRNA levels were normalized relative to the U6 expression levels. The results are expressed as the means. Primer sequences used in this study are shown in Supplementary Table 6 . Bisulphite sequencing and MSP Genomic DNA was extracted from gastric biopsy tissue sections and subjected to sodium bisulphite modification using EpiTect Bisulfite Kits (Qiagen) following the manufacturer’s protocols. For bisulphite sequencing, sodium bisulphite-treated DNA was PCR amplified using primers common to methylated and unmethylated DNA sequences. The purified PCR products were separated into the Hp-infected and -uninfected groups. The mixed PCR products in each group were cloned into the pGEM-T Easy vector (Promega), and over 40 clones were sequenced. For MSP, the methylated and unmethylated human DNA obtained from the EpiTect PCR Control DNA Set (Qiagen) was used to generate methylation-specific primers and PCR annealing temperatures that specifically amplify only methylated or unmethylated DNA. Quantitative SYBR Green MSP was performed to determine the levels of miR-210 CpG DNA methylation using a LightCycler DX400 (Roche) and SYBR Premix Ex Taq II (TaKaRa). The DNA methylation levels of the miR-210 CpG island were calculated as the amount of methylated DNA relative to the total levels of methylated and unmethylated DNA. The primers, used in this study are listed in Supplementary Table 5 . In situ hybridization The tissues of Mongolian gerbils were dissected, fixed with Tissue Fixative (Genostaff), and then embedded in paraffin and sectioned at 5 μm. For in situ hybridization, tissue sections were de-waxed with xylene, and re-hydrated through an ethanol series and PBS. The sections were fixed with 4% paraformaldehyde in PBS for 15 min and then washed with PBS. The sections were treated with 8 μg ml −1 Proteinase K in PBS for 30 min at 37 °C, washed with PBS, re-fixed with 4% paraformaldehyde in PBS, again washed with PBS and placed in 0.2 N HCl for 10 min. After washing with PBS, the sections were acetylated by incubation in 0.1 M tri-ethanolamine-HCl, pH 8.0, 0.25% acetic anhydride for 10 min. After washing with PBS, the sections were treated with or without PBS at 80 °C for 5 min. Hybridization was performed with probes (miRCURY LNA microRNA Detection Control probe, miRCURY LNA miR-210 Detection probe (EXIQON) or Mongolian gerbils STMN1 detection probe) at 50 °C for 16 h. After hybridization, the sections were washed in 5 × HybriWash (Genostaff), equal to 5 × SSC, at 50 °C for 20 min and then in 50% formamide, 2 × HybriWash at 60 °C, followed by RNase treatment in 50 μg ml −1 RNaseA in 10 mM Tris-HCl, pH 8.0, 1 M NaCl and 1 mM EDTA for 30 min at 37 °C. Then the sections were washed twice with 2 × HybriWash for 20 min, twice 0.2 × HybriWash for 20 min and once with Tris-buffered saline with 0.1% Tween20 (TBST). After treatment with 0.5% blocking reagent (Roche) in TBST for 30 min, the sections were incubated with anti-DIG AP conjugate (Roche) diluted 1:1,000 with TBST for 2 h at room temperature. The sections were washed twice with TBST and then incubated in 100 mM NaCl, 50 mM MgCl 2 , 0.1% Tween 20, 100 mM Tris-HCl, pH 9.5. Colour reactions were performed with nitro-blue tetrazolium chloride/5-bromo-4-chloro-3-indolyl phosphate p-toluidine salt (NBT/BCIP) solution (Sigma) overnight and then washed with PBS. The sections were counterstained with Kernechtrot stain solution (Mutoh) and mounted with CC/Mount (Diagnostic Biosystem). Images were acquired from the stained specimens using a Micro Imager.M1 microscope (Carl Zeiss), Zeiss AxioVision and MosaiX Softwares. Immunofluorescence microscopy Anguilla anguilla agglutinin (AAA; Sigma-Aldrich) was Cy3 labelled using Cy3 monofunctional reactive dye (Amersham Bioscience). Immunofluorescence staining was performed as described previously (Mimuro et al. 2007). For PCNA staining, acetone-fixed sections were stained with anti-PCNA antibody (Santa Cruz, sc-56, 1:50 dilution) after epitope retrieval by heating in citrate buffer (10 mM sodium citrate buffer (pH 6.0)). Fluorescein Isothiocyanate-conjugated secondary antibody (Sigma, F2012, 1:100 dilution) was used to visualize mouse antibody. Cy3-labelled AAA was used to visualize pit cells. The stined specimens were examined with a confocal laser-scanning microscope (LSM510; Carl Zeiss) equipped with LSM510 version 3.2 software (Carl Zeiss). Statistical analysis Differences between groups in the experiments were assessed using the paired, two-tailed Student’s t -test. The data in Fig. 1b–d , Fig. 2c , Fig. 5 and 6a ; Supplementary Fig. 4 were statistically analysed using the Mann−Whitney U -test for unpaired groups. The other data were statistically analysed using Student’s t- test. How to cite this article: Kiga, K. et al. Epigenetic silencing of miR-210 increases the proliferation of gastric epithelium during chronic Helicobacter pylori infection. Nat. Commun. 5:4497 doi: 10.1038/ncomms5497 (2014).